A regulatory role forStaphylococcus aureustoxin–antitoxin system PemIKSa Toxin–antitoxin systems were shown to be involved in plasmid maintenance when they were initially discovered, but other roles have been demonstrated since. Here we identify and characterize a novel toxin–antitoxin system ( pemIK Sa ) located on Staphylococcus aureus plasmid pCH91. The toxin (PemK Sa ) is a sequence-specific endoribonuclease recognizing the tetrad sequence U↓AUU, and the antitoxin (PemI Sa ) inhibits toxin activity by physical interaction. Although the toxin–antitoxin system is responsible for stable plasmid maintenance our data suggest the participation of pemIK Sa in global regulation of staphylococcal virulence by alteration of the translation of large pools of genes. We propose a common mechanism of reversible activation of toxin–antitoxin systems based on antitoxin transcript resistance to toxin cleavage. Elucidation of this mechanism is particularly interesting because reversible activation is a prerequisite for the proposed general regulatory role of toxin–antitoxin systems. Toxin–antitoxin (TA) systems were initially characterized as components of low copy number plasmids, which ensured their stable maintenance [1] , [2] . It was established that daughter cells that lose the plasmid are selectively eliminated by the deleterious activity of the long half-life toxin, as the pool of labile antitoxin rapidly diminishes in the absence of synthesis of new molecules. However, the later discovery of TA systems located on bacterial chromosomes initiated a still largely unsettled debate concerning the broader biological role of TA systems [1] , [3] , [4] , [5] , [6] . It is currently thought that TA systems have a general role in regulation of the stress response. Recent studies have demonstrated great diversity among TA systems. Different systems sense diverse stimuli, and act as global regulators of gene expression. Under favourable growth conditions genes of most TA systems are coexpressed and the deleterious activity of the toxin is prevented by the antitoxin [7] . However, various stress stimuli alter the toxin/antitoxin balance, usually by inducing increased proteolytic degradation of the labile antitoxin [8] , [9] , [10] . The activated toxin induces a dormant state or other adaptations that enable the bacteria to survive environmentally unfavourable conditions [11] , [12] , [13] . However, it is unclear how the bacteria recover from this state, although it is evident that the ability to return to equilibrium is a prerequisite in an efficient regulatory system. This important issue was addressed in our study. Class II TA systems include toxins characterized by ribonucleolytic activity. Nonspecific ribonuclease toxins degrade total cellular RNA; their potential regulatory role is limited to cell growth inhibition (dormancy), with prolonged activation of these toxins leading to cell death (plasmid maintenance). However, many class II toxins are sequence-specific ribonucleases. For example, the MazF toxin from Escherichia coli hydrolyses mRNA at the A↓CA sequence [14] , where the arrow denotes the site of hydrolysis; the MazF homologues MazF-mt3, MazF-mt7, MazF Sa and MazF-cd from Mycobacterium tuberculosis , S. aureus and Clostridium difficile recognize pentad target sequences (UU↓CCU or CU↓CCU, U↓CGCU, U↓ACAU and U↓A↓C↓AU, respectively) [15] , [16] , [17] ; whereas MazF-hw from Haloquadra walsbyi recognizes seven consecutive nucleotides (UU↓ACUCA) [18] . The activity of highly sequence-specific toxins leads to selective degradation and, as a result, inhibition of translation from only a limited pool of transcripts; this process is termed RNA interference [19] , and probably constitutes an efficient means of global regulation of gene expression. TA-driven RNA interference has been implicated in the regulation of virulence and antibiotic resistance in numerous pathogens including M. tuberculosis [16] , S. aureus [15] , [20] , Yersinia pestis [21] , Helicobacter pylori [22] , Streptococcus mutans [23] and C. difficile [17] , and also among enterococci [24] . However, the occurrence of this mechanism remains largely speculative, and the very attractive concept of global regulation of virulence factor expression by TA systems in pathogenic bacteria still awaits thorough experimental characterization. Here we describe a novel TA system PemIK Sa in S. aureus CH91 and demonstrate that the toxin PemK Sa is a sequence-specific ribonuclease while the antitoxin PemI Sa inhibits the toxin by physical interaction. We show that the system efficiently maintains plasmids, but argue that nonrandom distribution of toxin target sequences in the staphylococcal transcriptome supports the concept of TA system regulation of gene expression and provide experimental examples of such regulation. Moreover, we propose a possible mechanism of reversible activation of TA systems, which is indispensible for the postulated regulatory role of PemIK Sa and other similar systems. S. aureus plasmid pCH91 encodes a toxin–antitoxin system We identified a putative TA system encoded on S. aureus plasmid pCH91. The putative toxin (PemK Sa ; 112 amino acids) and the putative antitoxin (PemI Sa ; 89 amino acids) were encoded by the SACH_a18 and SACH_a19 loci, respectively. To verify the predicted function of those proteins, the respective coding sequences (CDSs) were cloned into the expression plasmids pETDuet-pemK Sa and pETDuet-pemI Sa . Expression plasmid pACYCDuet-pemI Sa , which is compatible with pETDuet, was also constructed. Furthermore, plasmid pETDuet-pemIK Sa was prepared where pemK Sa and pemI Sa were cloned under the control of two independent T7 promoters. Upon induction with isopropyl-β-D-thiogalactoside (IPTG), E. coli BL21(DE3) carrying pETDuet-pemI Sa expressed large quantities of His 6 -PemI Sa , as evidenced by SDS–polyacrylamide gel electrophoresis (PAGE) ( Fig. 1a and Supplementary Fig. S1 ). Protein expression was not observed from pETDuet-pemK Sa under comparable experimental conditions. Rather, IPTG induction resulted in growth inhibition ( Supplementary Fig. S2 ) while coexpression of PemI Sa from pACYCDuet-pemI Sa restored the production of PemK Sa . A similar effect occurred when both proteins were coexpressed from pETDuet-pemIK Sa , which indicates that PemI Sa eliminated the toxicity of PemK Sa to the host; thus, PemIK Sa exhibits characteristics of a typical TA system. 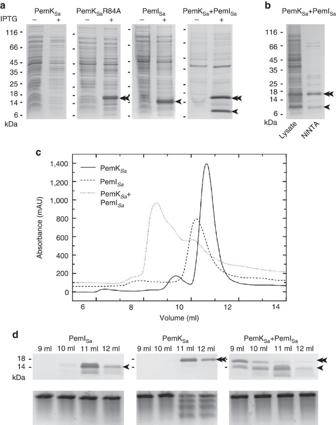Figure 1: Basic properties of the components of the PemIKSatoxin–antitoxin system. (a) Coexpression of PemISarestored the accumulation of PemKSa. SDS–PAGE of total cell lysates ofE. coliBL21(DE3) carrying plasmids driving the expression of His6-PemKSa(toxin), His6-PemKSaR84A mutant, His6-PemISa(antitoxin), and coexpression of PemISaand His6-PemKSa. Recombinant protein production was induced with IPTG as indicated. Bands corresponding to PemISaand PemKSa(or PemKSaR84A) are marked with a single and a double arrowhead, respectively. (b) PemKSaand PemISaform complexesin vivo. His6-tagged PemKSawas coexpressed with native PemISa. Toxin was recovered from cell lysate by affinity binding and copurified proteins were analysed by SDS–PAGE. Arrowheads as in panela. (c)In vitrodemonstration of PemKSa–PemISacomplex formation. Purified components of the TA system were subjected to gel filtration separately or after mixing (using approximately a 1.5 molar excess of the antitoxin). (d) Analysis of fractions from gel filtration. SDS–PAGE of selected fractions (top), and agarose gel analysis of the effect of particular fractions on MS2 phage RNA (bottom). Only PemKSa(double arrowhead) but not PemISa(single arrowhead; the bands below that corresponding to PemISarepresent degradation products of labile antitoxin) or the PemKSa–PemISacomplex exhibited ribonucleolytic activity against MS2 RNA. Figure 1: Basic properties of the components of the PemIK Sa toxin–antitoxin system. ( a ) Coexpression of PemI Sa restored the accumulation of PemK Sa . SDS–PAGE of total cell lysates of E. coli BL21(DE3) carrying plasmids driving the expression of His 6 -PemK Sa (toxin), His 6 -PemK Sa R84A mutant, His 6 -PemI Sa (antitoxin), and coexpression of PemI Sa and His 6 -PemK Sa . Recombinant protein production was induced with IPTG as indicated. Bands corresponding to PemI Sa and PemK Sa (or PemK Sa R84A) are marked with a single and a double arrowhead, respectively. ( b ) PemK Sa and PemI Sa form complexes in vivo . His 6 -tagged PemK Sa was coexpressed with native PemI Sa . Toxin was recovered from cell lysate by affinity binding and copurified proteins were analysed by SDS–PAGE. Arrowheads as in panel a . ( c ) In vitro demonstration of PemK Sa –PemI Sa complex formation. Purified components of the TA system were subjected to gel filtration separately or after mixing (using approximately a 1.5 molar excess of the antitoxin). ( d ) Analysis of fractions from gel filtration. SDS–PAGE of selected fractions (top), and agarose gel analysis of the effect of particular fractions on MS2 phage RNA (bottom). Only PemK Sa (double arrowhead) but not PemI Sa (single arrowhead; the bands below that corresponding to PemI Sa represent degradation products of labile antitoxin) or the PemK Sa –PemI Sa complex exhibited ribonucleolytic activity against MS2 RNA. Full size image PemK Sa and PemI Sa physically interacted inside the cell, as PemI Sa was copurified from the cell lysate using His 6 -PemK Sa ( Fig. 1b and Supplementary Fig. S1 ). Indeed, purified PemI Sa forms a heterodimer with purified PemK Sa , as evidenced by gel filtration ( Fig. 1c and Supplementary Figs S3 and S4 ). PemK Sa -induced growth inhibition was partially reversed by a R84A mutation. Growth inhibition was still evident following induction of mutant production, but was not as pronounced as in the case of wild-type PemK Sa ( Supplementary Fig. S2 ). Moreover, mutant production was detectable in cell lysates using SDS–PAGE, whereas accumulation of the wild-type was not detected under similar conditions ( Fig. 1a ). This suggests that the deleterious effect of PemK Sa R84A was reduced but not completely eliminated. PemIK Sa system allows stable plasmid maintenance To investigate the stability of pCH91 in S. aureus strain CH91 the bacterium was subjected to cultivation under conditions known to cure bacteria of plasmids (4 °C, 42 °C, ultraviolet radiation). The presence of pCH91 was monitored using the reporter activity of staphopain C, a cysteine protease naturally overproduced from pCH91 (ref. 25 ). Under no tested conditions was the reporter activity reduced during the course of experiment (14 days), which indirectly suggests strong internal selective pressure for pCH91 maintenance. To determine whether PemIK Sa mediates plasmid stability, E. coli cells were cotransformed with pETDuet-pemK Sa and pACYCDuet-pemI Sa , and the stability of pACYCDuet-pemI Sa was monitored during cultivation in the presence of selective antibiotic pressure towards pETDuet-pemK Sa but not pACYCDuet-pemI Sa ( Supplementary Fig. S5 ). We assumed that if PemI Sa is essential to overcoming the deleterious activity of PemK Sa , then pACYCDuet-pemI Sa would stably propagate despite the absence of external selective antibiotic pressure. Indeed, pACYCDuet-pemI Sa was maintained throughout the experiment (23 days), but was largely lost on day 23 when pETDuet-pemK Sa was substituted with an empty pETDuet control plasmid ( Fig. 2a ). 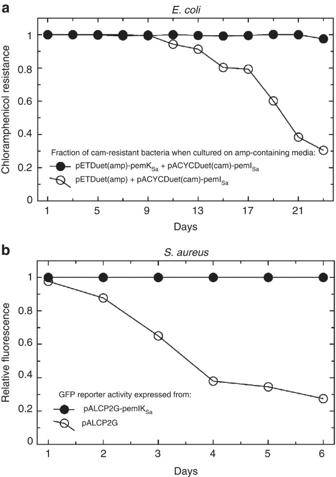Figure 2: PemIKSasystem maintains plasmid stability inE. coliandS. aureus. (a)E. coliwas cotransformed either with the PemISaexpressing and chloramphenicol resistance (cam) providing pACYCDuet-pemISaplasmid, and the PemKSaexpressing and ampicillin resistance (amp) providing pETDuet-pemKSaplasmid (filled circles), or pACYCDuet-pemISaand empty pETDuet (empty circles). The cells were cultured in the presence of ampicillin, and the stability of pACYCDuet (chloramphenicol resistance) was monitored. Only in the presence of PemKSawas the PemISa-encoding plasmid stably maintained. (b)S. aureuswas transformed with pALCP2G-pemIKSa(filled circles), a GFP-expressing reporter plasmid containingpemIKSaunder the control of its native promoter, or empty pALCP2G (empty circles). The cells were cultured in the absence of selective antibiotic, and plasmid stability was monitored by virtue of GFP reporter activity. Only thepemIKSa-containing but not the empty plasmid was stably maintained. Both panels: representative results of two independent experiments. Figure 2: PemIK Sa system maintains plasmid stability in E. coli and S. aureus . ( a ) E. coli was cotransformed either with the PemI Sa expressing and chloramphenicol resistance (cam) providing pACYCDuet-pemI Sa plasmid, and the PemK Sa expressing and ampicillin resistance (amp) providing pETDuet-pemK Sa plasmid (filled circles), or pACYCDuet-pemI Sa and empty pETDuet (empty circles). The cells were cultured in the presence of ampicillin, and the stability of pACYCDuet (chloramphenicol resistance) was monitored. Only in the presence of PemK Sa was the PemI Sa -encoding plasmid stably maintained. ( b ) S. aureus was transformed with pALCP2G-pemIK Sa (filled circles), a GFP-expressing reporter plasmid containing pemIK Sa under the control of its native promoter, or empty pALCP2G (empty circles). The cells were cultured in the absence of selective antibiotic, and plasmid stability was monitored by virtue of GFP reporter activity. Only the pemIK Sa -containing but not the empty plasmid was stably maintained. Both panels: representative results of two independent experiments. Full size image To verify the plasmid maintenance function of the PemIK Sa system in a homologous host, we introduced the pemIK Sa cassette under control of its native promoter into the pALCP2G reporter plasmid constitutively expressing green fluorescent protein (GFP). S. aureus strain RN4220 containing the resulting pALCP2G-pemIK Sa was cultured in liquid media without selective antibiotic. Empty pALCP2G was used as a control. The presence of the plasmid was monitored on subsequent days using GFP fluorescence, and on the last day of the experiment by comparative quantitative plating on agar media containing and deprived of a selective antibiotic. Under these conditions, pALCP2G-pemIK Sa was stably maintained throughout the experiment (6 days), whereas control plasmid was largely eliminated ( Fig. 2b ). These data directly demonstrate the plasmid stabilizing role of the PemIK Sa system in S. aureus . PemK Sa is a sequence-specific RNase We investigated the mechanism of PemK Sa toxicity against the host. Incubation of phage MS2 RNA in the presence of purified PemK Sa resulted in RNA degradation, suggesting PemK Sa has ribonucleolytic activity. The degradation pattern was distinct (not smeared), suggesting that the ribonuclease activity of PemK Sa is sequence specific or secondary structure specific ( Fig. 1d ). We identified the sites of hydrolysis of MS2 RNA using a modified primer extension method [16] . The identified cleavage sites ( Supplementary Table S1 and Supplementary Fig. S6 ) defined a perfect consensus (U↓AUU) recognized and hydrolysed by PemK Sa . No other sites of hydrolysis were detected. Although there are a total of 10 UAUU sites in MS2 RNA (RefSeq accession no. NC_001417), only seven were hydrolysed by PemK Sa in our experiments, most probably because of steric occlusion of the remaining three sites ( Supplementary Table S1 ). We also purified the PemK Sa R84A mutant and assayed its ability to degrade MS2 RNA. The activity of PemK Sa R84A was estimated to be ~10% of that of the wild-type (a 10-fold excess of mutant was required to obtain digestion comparable to that obtained with wild-type PemK Sa ). Using primer extension experiments, we demonstrated that R84A mutation affects only the rate of hydrolysis, and not its specificity. Using an in vitro MS2 RNA digestion assay and purified proteins, we demonstrated that PemI Sa stoichiometrically inhibited the ribonuclease activity of PemK Sa at a 1:1 molar ratio. The activity of the PemK Sa R84A mutant was also stoichiometrically inhibited by PemI Sa , demonstrating that the mutation did not affect the TA interface. Nonrandom distribution of UAUU in S. aureus transcriptome Analysis of available genomic data demonstrated that, unlike pemIK Sa of strain CH91, homologous pemIK systems are almost exclusively chromosomal ( Supplementary Fig. S7 ). Therefore, we investigated whether plasmid maintenance was the only function of pemIK Sa . A nonspecific RNAse would clearly suffice for a process of elimination of daughter cells not inheriting the plasmid. On the other hand, a sequence-specific RNAse, such as PemK Sa could exert a global regulatory effect by degrading only a selected pool of transcripts, provided that the recognized sequences are organized in the transcriptome in a nonrandom fashion. To evaluate whether the latter was the case, we calculated the expected distribution of the UAUU sequence in mRNA, and compared this with the observed distribution in the transcriptome of S. aureus strain ED98. This strain was chosen for analysis because its genomic sequence is known (in contrast to strain CH91), and it carries a pCH91 related pAvX plasmid [26] coding a TA system identical to PemIK Sa . Statistically, the PemK Sa target sequence should appear every 77 bases, and thus should occur at least once in every gene. Among 2,689 open reading frames (ORFs) encoded in the genome of S. aureus ED98 we identified 121 ORFs in which the PemK Sa target sequence was either absent (56 ORFs) or present, but statistically underrepresented (65 ORFs; P ′≤0.01). Interestingly, this group of ORFs was composed of nonrandom transcripts, and contained a substantial number of transcripts encoding proteins implicated in virulence ( Supplementary Fig. S8 ). These included a transcription regulator Fur [27] ; delta-hemolysin [28] ; extracellular enzymes comprising metalloprotease, lipase and coagulase [29] ; and host protein-binding proteins including clumping factor A, von Willebrant factor-binding protein, fibronectin-binding protein, and serine–aspartate repeat proteins [30] (for a full list see Supplementary Data 1 ). We also identified 214 ORFs in which the PemK Sa target sequence was statistically overrepresented ( P ′≥0.99). The majority of transcripts in this group encoded transmembrane transporters ( Supplementary Fig. S8 and Supplementary Data 1 ). The nonrandom distribution of the PemK Sa target sequence in the staphylococcal transcriptome argues in favour of the hypothesis of a regulatory role for PemK Sa . The presence of the PemK Sa target sequence in an RNA molecule does not necessarily imply its hydrolysis, as the process may be sterically hindered by secondary structures, RNA-binding proteins and other factors. Therefore, we experimentally verified in vitro and in vivo the anticipated differential vulnerability of representative transcripts from the groups described above to PemK Sa degradation. In vitro , the stability of transcripts exposed to PemK Sa was monitored using electrophoresis. Expectedly, the more recognition sites were present in a particular mRNA, the more efficiently it was degraded by PemK Sa ( Fig. 3a and Supplementary Fig. S9 ). To further verify the correlation, we have synthesized ScpB encoding gene ( scpBalt ) in which all eight PemK Sa target sequences were replaced with sequences encoding identical amino acids, but using different codons. Such transcript was not affected by PemK Sa in vitro contrary to scpB transcript, which was efficiently degraded ( Fig. 3a ). Moreover, we have synthesized NrdR encoding gene ( nrdRalt ) in which we introduced nine UAUU sequences in a way, which did not affect the amino acid sequence of encoded protein. Such transcript was efficiently degraded by PemK Sa in vitro contrary to nrdR transcript, which was resistant to PemK Sa -mediated hydrolysis ( Fig. 3a ). 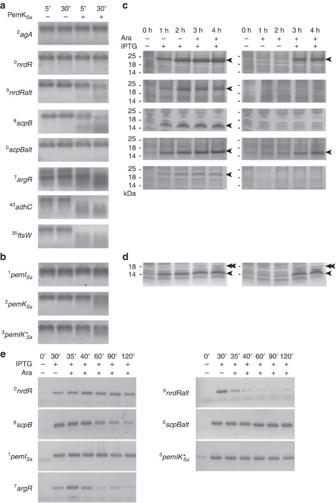Figure 3: PemKSamodulates gene expression by differentially targeting mRNA transcripts. (a) mRNA transcripts were incubated with PemKSafor the indicated time and analysed using agarose gel electrophoresis. The number of PemKSatarget sites (UAUU) in each transcript is denoted in superscript. Representative transcripts belonging to the groups where the PemKSatarget sequence is: underrepresented (agAandnrdR), overrepresented (adhCandfstW) or follows random distribution (scpBandargR) were chosen.scpBaltandnrdRaltare versions ofscpBandnrdRgenes where PemKSatarget sequences were removed and introduced, respectively. (b) Transcripts encoding PemISa, PemKSaand the whole, functionally deficientpemIKSa* transcript were treated with PemKSain vitro. Despite the presence of the PemKSatarget sequence in each transcript, no hydrolysis was observed inpemISa, whereas the toxin encoding part, as well as the wholepemIKSa* transcript were only inefficiently hydrolysed. (c) SDS–PAGE of total cell lysates ofE. coliBL21(DE3) cotransformed with arabinose inducible pBAD-pemKSaplasmid, and the respective IPTG inducible pACYCDuet-based plasmids. Single arrowheads indicate proteins expressed from pACYCDuet. Note that transcripts resistant to hydrolysis by PemKSa(a) drove expression of respective proteins in the presence of PemKSain vivo, while no expression occurred from transcripts susceptible to PemKSa. The timescale and major events are indicated at the top of the panel. (d) Experiment identical to that incsave that production of antitoxin was monitored (single arrowhead; toxin—double arrowhead). (e) Influence of PemKSaon the accumulation of transcripts expressed from pACYCDuet. At each indicated time point total cellular RNA was isolated, reverse transcribed and the amount of particular transcripts was analysed by PCR. Figure 3: PemK Sa modulates gene expression by differentially targeting mRNA transcripts. ( a ) mRNA transcripts were incubated with PemK Sa for the indicated time and analysed using agarose gel electrophoresis. The number of PemK Sa target sites (UAUU) in each transcript is denoted in superscript. Representative transcripts belonging to the groups where the PemK Sa target sequence is: underrepresented ( agA and nrdR ), overrepresented ( adhC and fstW ) or follows random distribution ( scpB and argR ) were chosen. scpBalt and nrdRalt are versions of scpB and nrdR genes where PemK Sa target sequences were removed and introduced, respectively. ( b ) Transcripts encoding PemI Sa , PemK Sa and the whole, functionally deficient pemIK Sa * transcript were treated with PemK Sa in vitro . Despite the presence of the PemK Sa target sequence in each transcript, no hydrolysis was observed in pemI Sa , whereas the toxin encoding part, as well as the whole pemIK Sa * transcript were only inefficiently hydrolysed. ( c ) SDS–PAGE of total cell lysates of E. coli BL21(DE3) cotransformed with arabinose inducible pBAD-pemK Sa plasmid, and the respective IPTG inducible pACYCDuet-based plasmids. Single arrowheads indicate proteins expressed from pACYCDuet. Note that transcripts resistant to hydrolysis by PemK Sa ( a ) drove expression of respective proteins in the presence of PemK Sa in vivo , while no expression occurred from transcripts susceptible to PemK Sa . The timescale and major events are indicated at the top of the panel. ( d ) Experiment identical to that in c save that production of antitoxin was monitored (single arrowhead; toxin—double arrowhead). ( e ) Influence of PemK Sa on the accumulation of transcripts expressed from pACYCDuet. At each indicated time point total cellular RNA was isolated, reverse transcribed and the amount of particular transcripts was analysed by PCR. Full size image To verify the ability of PemK Sa to differentially target transcripts in vivo, we have produced selected staphylococcal mRNAs in E. coli and evaluated their stability upon ectopic expression of PemK Sa . The stability of tested transcripts inversely correlated with the number of PemK Sa target sites and correlated with the stability determined in the in vitro experiments ( Fig. 3e and Supplementary Fig. S10 ). To confirm the above findings in the native host and further assess the possible effects of cellular factors, we have introduced PemK Sa -encoding gene under the control of inducible promoter (pCN51-pemK Sa ) into S. aureus RN4220. Induction of the PemK Sa production resulted in growth inhibition, both in liquid and on solid media, in comparison with the bacteria carrying empty plasmid ( Fig. 4a ). Total RNA was isolated at various time points after induction of the toxin expression and the relative amount of selected transcripts was assessed using reverse transcriptase PCR. Again, transcript stability inversely correlated with the number of PemK Sa target sequences. In case of a single transcript ( argR ) protection against PemK Sa mediated degradation was observed in S. aureus compared with E. coli model and the results obtained in vitro ( Fig. 4c and Supplementary Fig. S11 ). 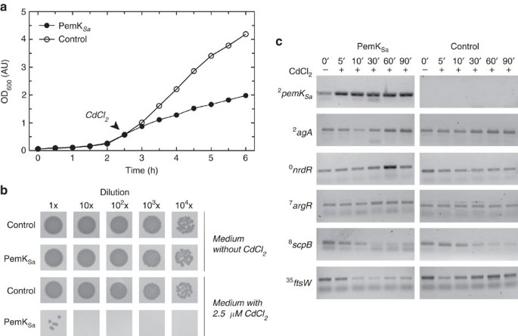Figure 4: PemKSainduces growth inhibition and selective transcript degradation inS. aureus. (a) Induction (CdCl2) of ectopic production of PemKSain the cell, results in growth inhibition ofS. aureusRN4220 in liquid medium. Representative results of two independent experiments. (b) Same as ina,but on solid media. The bacteria were diluted as indicated and plated on inducing (CdCl2) and non-inducing solid media. (c) Transcripts are differentially susceptible to PemKSainS. aureus. PemKSaexpression was induced and total mRNA was isolated at indicated time points. Level of indicated transcripts was assessed by reverse transcriptase PCR and electrophoretic analysis of reaction products.adhCwas transcriptionally silent, which did not allow to asses itsin vivostability (compare withFig. 3). All panels: Expression of PemKSawas driven from pCN51-pemKSawhile the control contained empty pCN51 plasmid only. Figure 4: PemK Sa induces growth inhibition and selective transcript degradation in S. aureus . ( a ) Induction (CdCl 2 ) of ectopic production of PemK Sa in the cell, results in growth inhibition of S. aureus RN4220 in liquid medium. Representative results of two independent experiments. ( b ) Same as in a, but on solid media. The bacteria were diluted as indicated and plated on inducing (CdCl 2 ) and non-inducing solid media. ( c ) Transcripts are differentially susceptible to PemK Sa in S. aureus . PemK Sa expression was induced and total mRNA was isolated at indicated time points. Level of indicated transcripts was assessed by reverse transcriptase PCR and electrophoretic analysis of reaction products. adhC was transcriptionally silent, which did not allow to asses its in vivo stability (compare with Fig. 3 ). All panels: Expression of PemK Sa was driven from pCN51-pemK Sa while the control contained empty pCN51 plasmid only. Full size image The above data collectively suggest that PemK Sa is capable of selectively targeting particular transcripts in the cellular pool of mRNA, possibly in a dose-dependent manner. As such, PemK Sa may function as a global regulator of S. aureus gene expression, downregulating the housekeeping metabolism and transmembrane transport while preserving the expression of selected virulence related genes. Return to equilibrium following temporary system activation If PemIK Sa has a regulatory function, mechanisms must exist to return the system to equilibrium following temporary activation. It is widely accepted that TA systems are induced by degradation of labile antitoxin, but there is no explanation for how, or whether, these systems return to equilibrium. We hypothesized that restoration of the equilibrium of temporarily activated PemIK Sa system is a self-perpetuating process dependent on the resistance of the antitoxin transcript to the ribonucleolytic activity of the toxin. PemI Sa - and PemK Sa -encoding transcripts contain one and two PemK Sa target sequences, respectively. However, when we treated the transcripts encoding the TA system components, PemI Sa and PemK Sa , or the whole pemIK Sa transcript, with purified toxin, the transcripts remained largely unaffected ( Fig. 3b and Supplementary Fig. S9 ) under conditions where susceptible transcripts (such as those of AdhC or FstW) were completely degraded ( Fig. 3a ). Significantly, the part of pemIK Sa transcript encoding the antitoxin was fully stable while that encoding the toxin was partially hydrolysed, but only inefficiently ( Fig. 3b ). Concurrently, computational modelling of the secondary structures of pemIK Sa mRNA demonstrated that all putative cleavage sites are located in double-stranded regions ( Supplementary Fig. S12 ), and are, therefore, inaccessible to PemK Sa . As ribosomes and RNA-binding proteins may alter higher-order mRNA structures, we have verified the stability of pemIK Sa transcript in vivo . To exactly define the time point of PemK Sa activation, its transcript was provided in trans while the analysed pemIK transcript ( pemIK Sa *) contained frameshifts in both PemI Sa and PemK Sa -encoding fragments, both resulting in premature termination of translation. When the pemIK Sa * transcript was challenged with ectopically expressed PemK Sa , only negligible decrease in the amount of the transcript was observed compared with other susceptible transcripts evaluated in the same conditions ( Fig. 3e ). This suggests that PemK Sa has no or only little effect on antitoxin translation, and in the absence of tertiary effects, the system should spontaneously return to equilibrium as soon as the stimulus that initially triggered the TA system imbalance is removed. To assess whether the antitoxin is continuously synthesized, or if the overall burden associated with toxin activation arrests cellular protein synthesis, sequential expression of PemK Sa and PemI Sa was attempted. E. coli was transformed with pBAD-pemK Sa and pACYCDuet-pemI Sa , the expression of recombinant toxin and antitoxin was sequentially induced, and the accumulation of both proteins was monitored. Consistent with other experiments in this study ( Supplementary Fig. S2 ), induction of toxin expression in the absence of antitoxin expression resulted in growth inhibition, and no toxin accumulation was detected. Induction of antitoxin production alone resulted in efficient expression. Simultaneous induction of PemI Sa and PemK Sa resulted in detectable expression of both proteins. Significantly, sequential induction of toxin followed by induction of antitoxin, even when separated by a period of 3 h, resulted in efficient translation of antitoxin ( Fig. 3d and SupplementaryFig. S13 ). This indicates that the protein synthesis apparatus remains functional long after toxin activity is induced. Further supporting this interpretation, recombinant NrdR (a transcript not affected by PemK Sa ) was expressed despite prior toxin induction, whereas no production of recombinant ArgR or ScpB (both transcripts are susceptible to PemK Sa ) was observed after induction of the toxin ( Fig. 3a ). To verify that inhibition of ScpB production upon PemK Sa induction is a direct effect of scpB transcript degradation by PemK Sa and not other tertiary effects we evaluated if scpBalt is capable to drive efficient expression of ScpB in the presence of PemK Sa . In vivo , ScpB protein was efficiently produced from scpBalt gene despite ectopic expression of PemK Sa ( Fig. 3c ). Conversely, no accumulation of NrdR protein was observed when nrdRalt was used instead of nrdR ( Fig. 3c ). Overall, the susceptibility of mRNA to the toxin determines the fate of particular protein synthesis upon TA system induction, whereas the protein translation apparatus remains functional. These results strongly support our hypothesis of self-perpetuating restoration of TA system equilibrium. The plasmid maintenance function of TA systems has been well established [1] , [2] , but increasing number of recent studies suggest a regulatory role of TA systems in broadly defined stress response [7] , [31] . Our current understanding of the latter function of TA systems is largely speculative, but if confirmed, TA systems are likely to emerge as one of the most versatile global regulatory systems in bacteria. Multiple chromosome-encoded TA systems have been identified [32] , and many of these contain site-specific ribonucleases. The low-specificity mycobacterial toxins MazF-mt1 (U↓AC) and MazF-mt6 (cleaves preferentially in U-rich regions) cause growth inhibition when heterologously expressed in E. coli , whereas MazF-mt3 (UU↓CCU, CU↓CCU) and MazF-mt7 (U↓CGCU) show almost no effect [16] , [33] . PemK Sa (U↓AUU) induces an intermediate effect when expressed in E. coli , inhibiting growth in liquid, but not on solid media. Although the above differential influence may be modulated by other factors (such as for example the level of overexpression), it seems reasonable to hypothesize that the longer the recognition sequence the greater the potential to selectively target only parts of the transcriptome. Importantly, although pemIK Sa was identified on a plasmid in strain CH91, almost identical systems are present throughout the Staphylococcus genus, and with only one exception are localized on the bacterial chromosome ( Supplementary Fig. S7 ). This suggests that the system may be transmitted between the chromosome and plasmids, but also that its primary role is distinct from plasmid maintenance. Several studies have demonstrated that recognition sequences of particular interferases are distributed in a nonrandom fashion in the transcriptome of host species. This suggested that bacterial genomes have coevolved with interferases to distinguish susceptible and resistant gene pools, and thus facilitate global regulation. Only simple models, based on frequencies of particular nucleotides in all CDSs, have previously been used to predict the expected random distribution of interferase target sequences in the transcriptome [14] , [16] , [34] . Comparison with the observed distribution enabled groups of transcripts with significantly underrepresented or overrepresented interferase recognition sequences to be distinguished. Here we proposed a more biologically relevant model based on frequencies of coding triplets. Our model provides predictions that better fit the observed distribution, and limits the number of sequences outside the assumed confidence interval, which enables better prediction of the pools of transcripts likely to be differentially regulated by the interferase ( Supplementary Fig. S14 ). It is of note that for the tested interferases these pools of transcripts are surprisingly functionally consistent. For example, the MazF-mt3 or MazF-mt7 recognition sequence is underrepresented in a subset of genes of the PE and PPE families, which are important in the immunopathogenicity of M . tuberculosis [16] . Further, the recognition sequence for MazF-cd is underrepresented in toxB and cwpV genes, encoding factors implicated in virulence [17] . We argue that PemIK Sa is involved in virulence modulation in S. aureus , based on the fact that the PemK Sa recognition sequence is underrepresented in a range of genes encoding virulence factors. As the MazF Sa toxin has also been implicated in regulation of staphylococcal virulence [15] , interferase-mediated modulation of virulence factors emerges as a common trait. Another large group of transcripts potentially regulated by PemK Sa includes those encoding transmembrane transporters. This is consistent with other studies arguing that not only groups of genes related to virulence are potentially susceptible to TA-mediated regulation (although some transmembrane transporters are involved in pathogenesis). For example, in the soil bacterium Bacillus subtilis a group of transcripts encoding proteins involved in antibiotic synthesis has been predicted to be resistant to MazF Bs , based on statistical analysis [35] . Although the specificities of MazF Bs , MazF Sa and MazF-cd are identical, the range of affected transcripts differs. This clearly indicates adaptive evolution of the genomes to differentially exploit the regulatory potential of similar interferases among different species. Although computational analyses consistently demonstrate functionally related pools of transcripts as being potentially resistant/susceptible to interferase action, the regulatory function of interferases remains a tempting hypothesis rather than a proven fact. The experimental evidence concerning the presumed regulatory role of TA interferases is almost nonexistent. Most significantly, the differential susceptibility of four different transcripts to MazF Sa has been demonstrated. mRNA encoding pathogenic adhesive factor SraP was rapidly degraded by MazF Sa (ref. 15 ), whereas transcripts of housekeeping genes (including recA , gyrB and sarA ) were resistant [34] . This is the only previous direct experimental demonstration of TA-mediated regulation of transcript stability we are aware of. Thus, our comprehensive demonstration of a direct correlation between the predicted and observed susceptibility of different transcripts to interferase in vitro , and the observation that resistant, but not susceptible transcripts are able to drive the expression of their respective proteins in vivo despite activation of the TA system, strongly support the proposed regulatory function of TA systems. Given the recent speculation about the regulatory role of TA systems, it is surprising that no consistent model of their reversible activation has been provided. It is generally accepted that TA systems are activated in response to external stimuli. However, regulatory function requires both an activating mechanism and an efficient means of switching between the active and inactive states. Although obvious, this requirement has never previously been comprehensively investigated with respect to TA systems. In this study, we hypothesized and provided experimental verification that a TA system returns to homoeostasis by virtue of a self-perpetuating process. According to our model, in homoeostasis the entire pool of toxin remains associated with the antitoxin. An external stimulus induces degradation of labile antitoxin, thus releasing the toxin activity. As the transcript encoding the antitoxin is resistant to interferase, the antitoxin is constitutively produced despite system activation. As soon as the activating stimulus ceases, the antitoxin accumulates and the system returns to equilibrium ( Fig. 5 ). This model predicts gradual toxin activation dependent on the strength of the stimulus, which is noteworthy in view of the demonstrated differential susceptibility of toxin-sensitive transcripts. 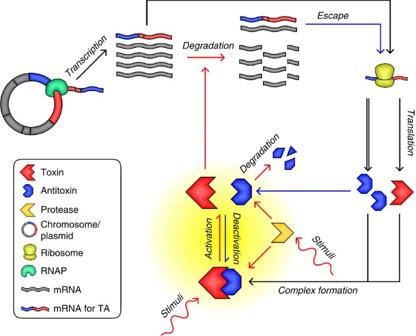Figure 5: Proposed mechanism of reversible activation of type II TA systems. In homoeostasis the toxin remains neutralized by the antitoxin. An external stimulus depletes the antitoxin, releasing the ribonucleolytic activity of the toxin. Antitoxin mRNA and translation machinery are insensitive to the toxin. As soon as the stimulus ceases, the antitoxin turnover slows down, and the system returns to equilibrium. Black arrows: normal growth conditions, TA system inactive or processes independent of TA system activation. Red arrows: TA system activation in response to external stimulus. Blue arrows: processes leading to TA system deactivation. Note: the nature of the stimulus and its target(s) are currently unknown. Figure 5: Proposed mechanism of reversible activation of type II TA systems. In homoeostasis the toxin remains neutralized by the antitoxin. An external stimulus depletes the antitoxin, releasing the ribonucleolytic activity of the toxin. Antitoxin mRNA and translation machinery are insensitive to the toxin. As soon as the stimulus ceases, the antitoxin turnover slows down, and the system returns to equilibrium. Black arrows: normal growth conditions, TA system inactive or processes independent of TA system activation. Red arrows: TA system activation in response to external stimulus. Blue arrows: processes leading to TA system deactivation. Note: the nature of the stimulus and its target(s) are currently unknown. Full size image We experimentally demonstrated that all the requirements necessary for the proposed mechanism to function were fulfilled. First, we showed that the pemIK Sa transcript was relatively resistant to PemK Sa compared with other, susceptible genes. Second, we demonstrated that PemK Sa -associated RNA interference did not directly affect the cell translation machinery, which remained functional despite toxin activation. Third, we showed that PemI Sa was expressed even in the presence of active toxin. A simple mechanism such as that described here could potentially regulate all TA systems where the toxin is a sequence-specific RNAse. Indeed, the pentad sequences recognized by MazF-mt3, MazF-mt7, MazF Sa , MazF Bs and MazF-cd are absent in the transcripts of their respective antitoxins [15] , [16] , [17] , [35] . Moreover, toxins other than PemK Sa do not interfere with cell translation machinery [17] , [36] . Currently, the most important question remaining is whether global analyses of interferase effects on transcriptomes and proteomes will confirm the assumptions concerning their universal regulatory role in bacteria. Bacterial strains and culture conditions E. coli strains DH5α and BL21(DE3) were cultured in Luria broth (LB). S. aureus strains CH91 and RN4220 were grown in tryptic soy broth. All cultures were incubated at 37 °C with thorough aeration. For plasmid propagation, the media were supplemented with ampicillin (amp) (100 μg ml −1 ) or chloramphenicol (cam) (34 μg ml −1 and 10 μg ml −1 for E. coli and S. aureus , respectively). Plasmid constructs Standard molecular biology techniques were used in the construction of plasmids [37] . The pemI Sa and pemK Sa were amplified from plasmid pCH91 (GenBank: JQ619831 ), which was isolated form S. aureus CH91 (ref. 38 ). agA , nrdR , adhC and fstW were amplified from the chromosomal DNA of strain CH91. argR and scpB were amplified from genomic DNA of S. aureus NCTC 8325. Amplicons were ligated into pTZ-57R/T (Fermentas), excised and transferred into target vectors: pACYC-Duet1, pETDuet1 (Novagen), pBAD-His/A (Invitrogen), pCN51 (ref. 39 ), and pALCP2G (this study). nrdRalt and scpBalt were synthesized de novo (Life Technologies, Supplementary Table S2 ) and cloned into the pACYC-Duet1. QuickChange Site-directed Mutagenesis Kit (Stratagene) was used for plasmid mutagenesis. The primer sequences and plasmids used in this study are summarized in Supplementary Tables S3 and S4 , respectively. Protein expression and purification Recombinant proteins were produced in E. coli BL21(DE3). Expression was induced with 1 mM IPTG. Six histidine tagged antitoxin PemI Sa was expressed from pETDuet-pemI Sa . A similarly tagged toxin mutant was expressed from pETDuet-pemK Sa R84A. Both proteins were recovered using affinity chromatography under native conditions. His 6 -tagged PemK Sa was coexpressed with native PemI Sa using pETDuet-pemIK Sa . PemK Sa was purified from the complex with PemI Sa using affinity chromatography in denaturing conditions, and refolded by dialysis against 50 mM sodium phosphate pH 8.0 containing 300 mM NaCl and 20% glycerol. For each protein, the final purification step consisted of gel filtration on Superdex 75 (GE Healthcare) in 50 mM sodium phosphate, pH 8.0 containing 100 mM NaCl (buffer GF). All preparations obtained were homogenous, as determined using SDS–PAGE [40] . Plasmid maintenance tests E. coli BL21(DE3) were double-transformed with pETDuet-pemK Sa and pACYCDuet-pemI Sa or pETDuet and pACYCDuet-pemI Sa , inoculated into LB supplemented with amp, and cultured overnight (ON). Each following day a new culture was set up by 1,000 times dilution of the ON culture into fresh LB with amp. Simultaneously, the aliquot of bacteria was diluted and plated on LB agar with amp. Colonies were counted and transferred on LB agar with amp and cam using replica plate method [41] . The percentage of cam resistant colonies relative to amp resistant colonies was determined. S. aureus RN4220 was transformed either with pALCP2G-pemIK Sa or empty pALCP2G, inoculated to tryptic soy broth with no selective antibiotic, and incubated ON. Subsequent cultivation was performed as described above, save that bacteria were plated on tryptic soy broth agar and the percentage of colonies that retained the ability to express GFP was determined. On the last day of the experiment, the percentage of colonies resistant to cam relative to all colonies was determined by replica plate method. Assessment of RNA hydrolysis sites by primer extension The total RNA of phage MS2 was reacted with PemK Sa according to the protocol of Zhu et al. [16] , with the exception that the RNA chaperone CspA was not included. Briefly, 1 μg of MS2 RNA and 10 pmol of PemK Sa were incubated at 37 °C in 10 mM Tris-HCl (pH 8.0) containing 10 mM EGTA in a total volume of 10 μl for 30 min. Primer extension was performed as described by Nadratowska-Wesolowska et al. [42] with slight modifications. Briefly, toxin-digested MS2 RNA was mixed with 0.5 pmol of 32 P-labelled primer ( Supplementary Table S5 ), incubated for 20 min at 70 °C, then slowly cooled to 40 °C and transferred to an ice bath. M-MuLV buffer, deoxyribonucleotide triphosphates, RevertAid M-MuLV Reverse Transcriptase and RNase inhibitor (Fermentas) were added. The reaction was continued for 60 min at 42 °C, and terminated by addition of denaturing solution (95% formamide, 10 mM EDTA, 0.1% xylene cyanol, 0.1% bromophenol blue) and incubation at 70 °C for 5 min. The reaction products were separated by electrophoresis in 8% polyacrylamide gel containing 8 M urea, and the bands were visualized on X-ray film. Coexpression assay Bacteria were grown in LB containing selection antibiotics to optical density at 600 nm (OD 600 ) ~0.5 before induction of recombinant proteins expression. In case of pETDuet-pemK Sa and pACYCDuet-pemI Sa cotransformants, the expression from both plasmids was induced simultaneously with IPTG. In case of pBAD-pemK Sa carrying cotransformants, PemK Sa expression was induced with arabinose and partner coexpression was induced with IPTG at time points indicated on Fig. 3c . Expression of recombinant proteins were analysed by SDS–PAGE. In vitro PemIK Sa complex formation Samples containing 30 nmol of PemK Sa , 45 nmol of PemI Sa or mixture of above were analysed by gel filtration using the Superdex 75 HR column (GE Healthcare) in buffer GF. Fractions were analysed by SDS–PAGE and MS2 RNA degradation assay. Bioinformatic analysis The probability ( P ) of finding K interferase recognition sequence(s) in a CDS of length L can be calculated using the binominal distribution according to equation 1: where n is the number of sites where a super-motif of length l ′ (containing an interferase recognition sequence of length l ) can be placed in the CDS, according to equations 2 and 3: note that biologically meaningful L values are multiples of three. The super-motifis defined as the smallest number of sequential codons necessary to accommodatethe interferase recognition sequence in all three possible positions with respect toan open reading frame ( Supplementary Fig. S14 ). The total probability ( p tot ) of finding the interferase recognition sequence along the super-motif is related to the frequency of particular codons ( π i ). The frequency of codons in mRNA of S. aureus strain ED98 was determined based on all CDSs in GenBank records CP001781 , CP001782 , CP001783 and CP001784 . To avoid bias, the initial and stop codonswere omitted from the calculations. CDS of S. aureus ED98 were separated into three groups according to the distribution of interferase recognition sequences. Group I included transcripts where the interferase recognition sequence was strongly underrepresented ( P ′<0.01; equation 4) or absent. Group II contained transcripts that best fitted the probability distribution (0.01< P ′<0.99). Group III contained transcripts where the recognition sequence was strongly overrepresented ( P ′>0.99). The fitness of the resulting model was assessed by comparing the adjusted coefficient of determination based on sequence length standardized deviations with a similar coefficient calculated for the model based on nucleotide frequencies (the latter approach has been used by others to computationally assess the likely impact of mRNA interferases on the bacterial transcriptome [14] , [16] , [34] ). The internet tool implementing our model for analysis of user provided sequences is available at http://mol058.mol.uj.edu.pl/pemnetstat . All analysed genes were classified into three groups: ‘factors related to pathogenesis’, ‘transmembrane transporters’ and the remaining genes. Factors related to pathogenesis were annotated according to NCBI BioSystems database ( http://www.ncbi.nlm.nih.gov/biosystems ). This annotation was completed manually by referring to the literature. ‘Transmembrane transporters’ were assigned according to the annotation of S. aureus ED98 genome. Classification and annotation of genes are presented in Supplementary Data 1 . Susceptibility of staphylococcal mRNA to PemK Sa The mRNA of PemI Sa , PemK Sa and reporter proteins was obtained from the respective PCR amplified genomic sequences using TranscriptAid T7 High Yield Transcription Kit (Fermentas). In each case, 1 μg of mRNA was reacted with 10 pmol of PemK Sa at 37 °C for various time periods in 20 μl reaction mixture containing 10 mM Tris-HCl (pH 8.0) and 10 mM EGTA. The degree of hydrolysis was analysed using agarose gel electrophoresis. In vivo analysis of transcript levels Bacteria were collected at different time points from liquid culture by centrifugation. E. coli cells were resuspended in TRI Reagent. S. aureus cells were mechanically disintegrated in TRI using glass beads. Subsequent steps were performed using GeneJET RNA Purification Kit (Thermo Scientific). DNA contamination was removed with On-Column DNase I Digestion Set (Sigma-Aldrich). Complementary DNA was obtained using RevertAid Premium Reverse Transcriptase (Thermo Scientific) and random hexamers. In each case, 200 ng of total cellular RNA was used. PCR was carried out using the obtained complementary DNA and primers specific for each characterized gene ( Supplementary Table S3 ). The products were analysed by agarose gel electrophoresis in TAE buffer. How to cite this article: Bukowski, M. et al. A regulatory role for Staphylococcus aureus toxin–antitoxin system PemIK Sa . Nat. Commun. 4:2012 doi: 10.1038/ncomms3012 (2013).